On the conditions of magma mixing and its bearing on andesite production in the crust Mixing between magmas is thought to affect a variety of processes, from the growth of continental crust to the triggering of volcanic eruptions, but its thermophysical viability remains unclear. Here, by using high-pressure mixing experiments and thermal calculations, we show that hybridization during single-intrusive events requires injection of high proportions of the replenishing magma during short periods, producing magmas with 55–58 wt% SiO 2 when the mafic end-member is basaltic. High strain rates and gas-rich conditions may produce more felsic hybrids. The incremental growth of crustal reservoirs limits the production of hybrids to the waning stage of pluton assembly and to small portions of it. Large-scale mixing appears to be more efficient at lower crustal conditions, but requires higher proportions of mafic melt, producing more mafic hybrids than in shallow reservoirs. Altogether, our results show that hybrid arc magmas correspond to periods of enhanced magma production at depth. Although a strong case has been made for andesite arc magmas being by-products of basalt crystallization [1] , [2] , the generation of rocks of intermediate compositions has been also proposed to result from the juxtaposition and large-scale mixing of chemically contrasted magmas [3] , [4] , [5] , [6] , such as basalt and rhyolite [3] . Whether the latter is a general [3] , [4] or a subsidiary [7] process remains, however, debated. In the following, magma mixing is equivalent to hybridization and qualifies a homogeneous-looking mixture at the hand scale, whereas mingling represents an heterogeneous mixture whose two end-members can be clearly distinguished at the same, or higher, scale. Typically, magma mixing/mingling occurs during replenishment by a mafic magma of a felsic and mushy reservoir [8] , [9] , [10] , [11] , [12] , [13] , [14] , either deep or shallow, which, in the latter case, may trigger a volcanic eruption [8] . The injection of denser basalt into a lighter reservoir most likely produces viscous gravity currents spreading at the floor, leading to a stratified two-layer system [15] , except when excess momentum is available, which may induce fountaining [16] . Ensuing crystallization can lead to density inversion producing either local [17] , [18] or wholesale [19] overturning and associated mixing/mingling, depending on viscosity contrast [20] . Observations and fluid dynamical considerations [8] , [9] , [10] , [11] , [12] , [13] , [14] , [15] , [16] , [17] , [18] , [19] , [20] , [21] have shown that, in calcalkaline reservoirs, mixing/mingling most likely starts either from such boundary layer instabilities [17] , with centimetre to decimetre wavelength scale [18] , or from breakup of injected magma dykes [12] . These mechanisms readily explain enclave sizes as observed in plutonic or volcanic rocks [18] , [21] , that is, mingled magmas. However, a further step is required to shift from such a macroscopic heterogeneous rock to a homogeneous mixture at the hand scale, where mixing is revealed chiefly by the occurrence of several crystal populations [22] , [23] . It is this second step that we wish to address more specifically in our study. Previous work has considered magma mixing using analogical, numerical or experimental approaches [8] , [9] , [10] , [11] , [12] , [13] , [14] , [15] , [16] , [17] , [18] , [19] , [20] , which have all yielded valuable information on the fluid mechanics, leading to efficient stirring. However, the rigorous evaluation of the conditions favourable to intimate magma mixing has been hampered by the difficulty of simulating mixing at high pressure, and by the complex fluid-mechanical behaviour of magmas. In particular, the widely held assumption that mixing is feasible at low viscosity, contrasts only [9] , has not yet received experimental confirmation for real magmatic mixtures. In addition, early studies [9] , though paving the way for works such as the present one, did not have in hands precise phase equilibria of magmas under volatile-rich conditions, which are vital to constrain thermal exchange during mixing in arc settings. Laboratory work has concentrated mostly on mixing between silicate melts of contrasted viscosities [11] , and there have been no attempts to explore mixing under high-pressure conditions, which are necessary to dissolve volatiles into silicate liquids. To date, mixing with crystal-bearing silicate melts has been explored only at relatively fast strain rates, which are more appropriate to conduit flow conditions rather than those of reservoir, and the experiments were done at 1 bar, which prevented to investigate the role of volatiles [24] . We report here viscosity measurements performed during high-pressure felsic–mafic mixing experiments at moderate-to-low strain rates and P-T-fluid conditions relevant to crustal reservoirs [25] , [26] , [27] . These results are then combined with recent phase equilibria of magmas to evaluate the optimum conditions, leading to efficient mixing, that is, hybrids, when mafic and felsic magmas come into contact during single-intrusive events. We consider both lower and upper crust conditions, as mixing may occur at virtually all stages of magma evolution, either during emplacement in upper crust [28] , [29] , [30] , including before eruptions [31] , [32] , [33] , or in the deep crust [34] , [35] , [36] . In our modelling, we explore specifically the roles of mafic/felsic mass ratio, shear rate at the felsic–mafic interface and amount of gas, showing that mixing is promoted by higher values of any of these parameters. We consider our results in the context of the piecemeal nature of pluton growth [37] , [38] , which places stringent limits on the extent of mixing in shallow reservoirs, and conclude that hybrid andesites witness transient increase in mafic magma flux. Altogether, the calculations are used to infer how variations in magma supply rate may control magma mixing, hence the geochemical evolution of magma reservoirs through such a mechanism, and how it may ultimately affect continental crust evolution. High-pressure mixing experiments We performed torsion experiments on felsic–mafic-stacked layers, using an internally heated deformation apparatus [39] at conditions relevant to magmatic reservoirs in the upper crust ( P =300 MPa, T =600–1,200 °C, strain rates , magma viscosities=10 3 –10 12 Pa s, (refs 25 , 26 , 27 )). Before torsion experiments, we measured the viscosity of felsic and mafic end-members, which were found to agree with model predictions [40] . The torsion experiments involved fully molten and crystal-bearing felsic end-members and a crystal-bearing mafic magma. By changing the temperature, the crystallinity, hence viscosity, of the mafic material changed, so it was either more or less viscous than the felsic one. We considered that no mixing happened when the stack of layers with straight interfaces was preserved after deformation ( Fig. 1a ). In contrast, onset of mixing was characterized whenever interface instabilities-yielding mixing features similar to natural textures were observed ( Fig. 1b ). The geometry of the bulk deformation applied in all torsion experiments is that of simple shear, similar to that, which may occur at the vertical interface between a rising blob of magma through a more viscous one. In high-temperature runs, however, local departure from simple shear occurred, and a component of pure shear is probably present in some runs, as might happen on a top part of a rising blob of magma. Owing to technical limitations, the experiments did not allow us to apply very large amount of strain (γ), in particular at high temperature, which would have yielded homogeneous mixtures at the scale of our experimental samples (mm to cm) (when conditions appropriate to mixing were reached). Nevertheless, they document the incipient stages of magma mixing at the mm scale, illuminating, in particular, the important transition between unmixed and mixed regimes, where single crystals (or small clots of them) start to be detached from their parent magma and transported/embedded into foreign melt. We explored the juxtaposition and deformation of three pairs of magmas (see Supplementary Fig. 1 ): (1) dry dacite-haplotonalite, (2) dry basalt-haplotonalite and (3) hydrous basalt-haplotonalite (see Methods and Supplementary Fig. 1 ). 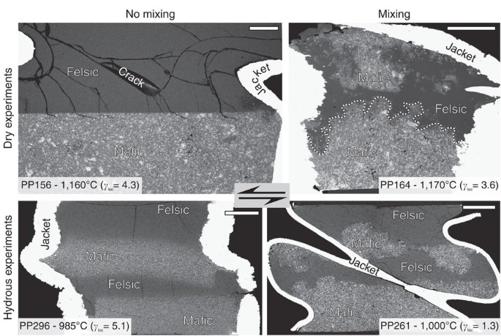Figure 1: Illustration of experimental textures. SEM images showing textures obtained when no mixing (a) and mixing (b) happen during torsion experiments on dry and hydrous samples. The felsic-mafic end-members are separated by a planar interface after torsion at 1,160 °C (or 985 °C for hydrous conditions), whereas complex textures develop at 1,170 °C (1,000 °C, hydrous) owing to interface instabilities and the collapse of the touching crystal framework in the mafic layer. Note the small temperature interval (<15 °C) over which such changes occur. Scale bars are 1 mm in PP156, PP296 and PP261, and 0.5 mm in PP164. Figure 1: Illustration of experimental textures. SEM images showing textures obtained when no mixing ( a ) and mixing ( b ) happen during torsion experiments on dry and hydrous samples. The felsic-mafic end-members are separated by a planar interface after torsion at 1,160 °C (or 985 °C for hydrous conditions), whereas complex textures develop at 1,170 °C (1,000 °C, hydrous) owing to interface instabilities and the collapse of the touching crystal framework in the mafic layer. Note the small temperature interval (<15 °C) over which such changes occur. Scale bars are 1 mm in PP156, PP296 and PP261, and 0.5 mm in PP164. Full size image The dry dacite-haplotonalite pair was deformed between 850 and 1,000 °C ( Fig. 2a ). In the temperature interval of 850–950 °C, despite the large amount of shear strain applied (γ up to 8) and a low viscosity contrast (log( η haplotonalite / η dacite )=0.3), no mixing occurred for viscosities in the range 10 12 –10 8 Pa s. Interface instability appeared only in the experiment conducted at 1,000 °C with the boudinage of the layers, corresponding to a measured viscosity of 10 7 Pa s. Hence, mixing of viscous and crystal-free melts, even differing little in viscosity, appears feasible at viscosities lower than 10 7.5 Pa s under the explored strain rates ( Fig. 2a ). 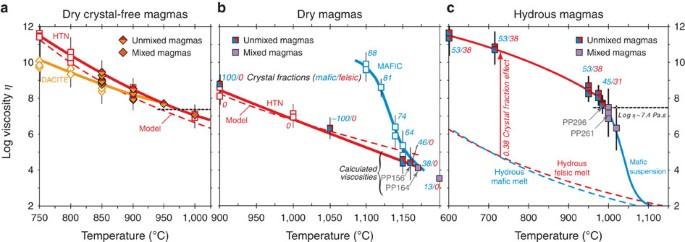Figure 2: Experimental magma viscosities during mixing. Measured viscosities versus temperature for the three pairs of magmas: dry dacite and haplotonalite (HTN) (a), dry basalt and haplotonalite (b) and hydrous basalt and haplotonalite (c). Half-filled symbols represent experiments where no mixing occurs (Fig. 1a), whereas filled symbols are those displaying mixing textures (Fig. 1b). Open symbols represent experiments performed on single end-members. Dashed red lines in (a) and (b) labelled “model” refer to ref.40model applied to end-member compositions. In panelsaandb, solid lines are hand-fitted trends to experimental data. In panel (c), dashed lines are melt viscosities calculated after ref.40, while blue/red solid lines are fitted by hand to experimental data. The vertical red arrow shows the calculated effect of 38% crystals. Italicized numbers next to each datum give the crystal fraction (blue-mafic and red-felsic). Error bars on measured viscosities are shown when larger than symbol size. In panelb, the lowest viscosities (around 104Pa s) were beyond reach of instrument capacities, and were calculated (see Methods). Figure 2: Experimental magma viscosities during mixing. Measured viscosities versus temperature for the three pairs of magmas: dry dacite and haplotonalite (HTN) ( a ), dry basalt and haplotonalite ( b ) and hydrous basalt and haplotonalite ( c ). Half-filled symbols represent experiments where no mixing occurs ( Fig. 1a ), whereas filled symbols are those displaying mixing textures ( Fig. 1b ). Open symbols represent experiments performed on single end-members. Dashed red lines in ( a ) and ( b ) labelled “model” refer to ref. 40 model applied to end-member compositions. In panels a and b , solid lines are hand-fitted trends to experimental data. In panel ( c ), dashed lines are melt viscosities calculated after ref. 40 , while blue/red solid lines are fitted by hand to experimental data. The vertical red arrow shows the calculated effect of 38% crystals. Italicized numbers next to each datum give the crystal fraction (blue-mafic and red-felsic). Error bars on measured viscosities are shown when larger than symbol size. In panel b , the lowest viscosities (around 10 4 Pa s) were beyond reach of instrument capacities, and were calculated (see Methods). Full size image The dry basalt-haplotonalite pair is characterized by a continuous decrease in viscosity contrast as temperature increases, owing to the increasing melt fraction of the mafic end-member ( Fig. 2b ). The viscosity contrast reaches its minimum at a temperature close to 1,170 °C, when both end-members have a viscosity of 10 4 Pa s ( Fig. 2b ). Deformation experiments reveal that this temperature is also the threshold for magma mixing: the initial stack geometry was preserved in the 600–1,160 °C temperature interval ( Fig. 1a ), during which all the strain was accommodated by the less viscous end-member, that is, the haplotonalite. We interpret this as the result of the high crystal fraction in the mafic end-member, which results in a continuous crystal network that increases the viscosity of the basalt ( Fig. 2b ), giving it a yield strength [41] , as long as the crystal fraction is higher than 46% (volume). At 1,170 °C, that is, only 10 °C higher, this touching crystal network collapses, decreasing the viscosity contrast between both end-members to log( η haplotonalite / η basalt )<0.5 ( Fig. 2b ), yielding mixing features similar to those observed in natural magmas, and which were observed in all experiments performed at 1,170 and 1,200 °C ( Fig. 1b ). The hydrous basalt-haplotonalite pair shows the effect of water on magma mixing. Before deformation, both end-members were annealed under hydrous conditions (see Methods). In the temperature interval 600–985 °C, corresponding to measured bulk viscosities between 10 12 –10 7.8 Pa s ( Fig. 2c ), no mixing was documented, all the deformation being accommodated again by the felsic layer ( Fig. 1a , lower panel). Mixing features were produced in experiments conducted at 1,000 °C ( Fig. 1b , lower panel), when the bulk viscosity was around 10 7.4 Pa s ( Fig. 2c ), and at higher temperatures. In all cases it occurred when the crystal fraction was lower than 45%, resulting in a small viscosity contrast (<0.5 log units), as observed under dry conditions ( Fig. 2b,c ). The role of water appears to be simply to decrease temperatures, which in the present case is shifted down by ~170 °C compared with dry conditions. The experiments document the fact that the transition between the no-mixing and mixing fields is sharp, occurring over <10 °C under dry conditions, and over ~15 °C with water ( Fig. 1 ), in both cases corresponding to a transition between locked to unlocked crystal network in the mafic end-member. Our results therefore reveal that, at shear rates expected to occur at depth [25] , [26] (<10 −3 s −1 ) mixing through enclave disaggregation is unlikely to occur if the mafic blob has a viscosity higher by >0.3 log unit relative to that of its host. Therefore, the fate of an enclave, that is, whether it disaggregates via lateral shearing or remains intact [42] , will be controlled by the viscosity contrast. The conditions for small viscosity contrast to be achieved are explored below but our experiments show that the amount of deformation required to disrupt the enclave into smaller parcels of magma or isolated crystals, is in all cases small (γ<4); hence, iso-viscous enclaves will disaggregate rapidly if strained along with the felsic host. Therefore, mafic enclaves preserved in felsic rocks most probably correspond to the case where the mafic blob was immersed into a felsic medium with a lower viscosity [43] . More generally, the experiments evidence that magma parcels having crystal contents higher than ~50% are sufficiently rigid to resist magmatic shear imposed by the background flow field, behaving like solid rather than liquid. The lack of mixing in the first series of deformation experiments (between haplotonalite and dacite melts) at viscosities higher than 10 7 Pa s may be related to the lack of crystals in either magmas. Occurrence of crystals likely affects the local stress field and possibly enhances mixing by triggering interface instabilities [24] . Relative masses of end-members These rheological constraints are now used to evaluate how contrasted pairs of natural magmas may well mix together. We have selected basalt, andesite, dacite and rhyolite compositions whose phase equilibria are known in the pressure range 0.2–1 GPa [44] , [45] , [46] , [47] , [48] , [49] , [50] . This allows us to establish the temperature-dependent crystal fraction ( Supplementary Fig. 2 ) and residual liquid composition, and in turn, to calculate the bulk viscosity of each magma at any temperature using an empirical model, which incorporates the effects of abundance and shape of crystals ( Fig. 3 , see Methods). 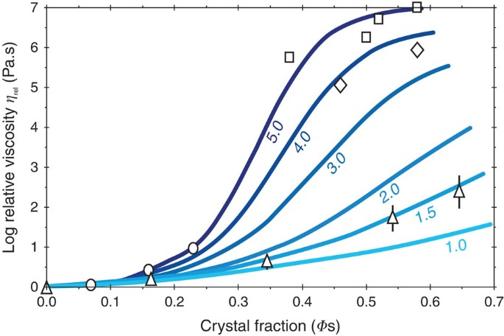Figure 3: Evolution of magma viscosity with crystal fraction and shape ratio. Each blue curve is labelled with the corresponding shape ratio of crystals. The calculations have been performed using the viscosity equation presented in Methods, which allows to incorporate the role of crystal shape, in addition to their abundance. Experimental magma viscosities obtained with different crystal shape ratios are shown along with calculated curves: open square: shape ratio=5; rhombus, shape ratio =3.5; circle, shape ratio= 4.9; triangle, shape ratio=1.5. Error bars on viscosity measurements are shown when greater than symbol sizes. Figure 3: Evolution of magma viscosity with crystal fraction and shape ratio. Each blue curve is labelled with the corresponding shape ratio of crystals. The calculations have been performed using the viscosity equation presented in Methods, which allows to incorporate the role of crystal shape, in addition to their abundance. Experimental magma viscosities obtained with different crystal shape ratios are shown along with calculated curves: open square: shape ratio=5; rhombus, shape ratio =3.5; circle, shape ratio= 4.9; triangle, shape ratio=1.5. Error bars on viscosity measurements are shown when greater than symbol sizes. Full size image Using the approach of ref. 9 , we calculated the thermal and rheological evolution of a system composed of two juxtaposed magmas, simulating the replenishment of a felsic reservoir by a hotter more mafic magma, for various fractions of mafic input, exploring a range of initial temperatures for the felsic end-member, whereas initial temperature of the mafic intrusive was near its liquidus. Typically, the cooling and associated crystallization of hydrous magmas, from basalt to rhyolite, result in the early increase of its viscosity ( Fig. 4 ). Figure 5 shows the cases when the initial felsic temperatures correspond to that of pre-eruptive storage temperatures, and the mafic end-member is an Mg-rich basalt. 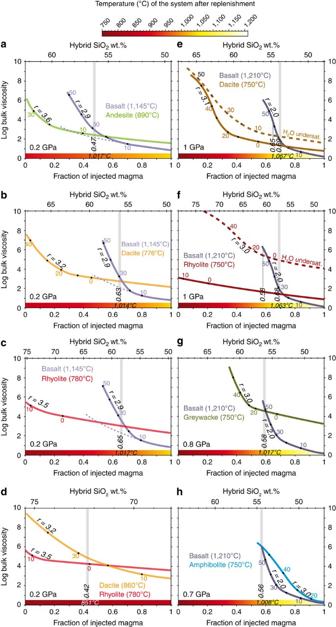Figure 5: Evolution of felsic and mafic magma viscosities with fraction of mafic magma. Viscosities are calculated for an average aspect ratio of crystals,r(given next to each curve) in each magma (seeFig. 3), and for the case of a hot mafic magma intruding either shallow (a,b,c,d) or deep (e,f,g,h) felsic reservoirs. Ticks on curves give the wt% of crystals of each end-member. The upper horizontal axis of each panel is graduated in terms of the SiO2(wt%) of the mixture corresponding to the mafic fraction. When the viscosity curves cross over, hybrid magmas are produced. Thick vertical grey lines indicate where the viscosity contrast is <5 (0.3 in log unit). The temperature of each felsic–mafic mixing pair is given by the colour-coded bars. The temperature of the hybrid corresponding to the minimum amount of mafic magma needed to reach near neutral viscosity contrast is given for each case. The initial temperature of magmas in each pair is given in parentheses next to composition. The thin-dashed lines extending the basalt curve on panelsa,bandcgive the expected bubble effect on viscosity (10% vol). Thick-dashed lines show the viscosity curves of H2O-undersaturated felsic magmas. In the case of an andesitic reservoir, magma mixing (that is, rocks formed where the felsic and mafic curves cross over or differ by >0.3 log units) happens when the mass of injected basalt almost equals the mass of the resident magma (0.47, Fig. 5a ). For more felsic reservoirs, dacitic or rhyolitic, the onset of mixing requires a larger mass fraction, respectively of 0.63 and 0.65 ( Fig. 5b,c ). Similarly, mixing with a colder (crystal-rich and near solidus) felsic end-member increases the minimum basalt proportions to beyond 0.7, leading to hotter hybrids ( Fig. 6a–c ). Using wet basalts as the mafic end-member increases the mafic fraction over 0.75 for both the dacite and rhyolite end-members ( Fig. 6d–f ). For the common case of andesite intruding a more felsic reservoir [24] , similar rheological patterns are observed ( Fig. 7 ), again implying large amounts of the more mafic magma for hybridization to proceed. Magma mixing is also sensitive to the mineral assemblage (influencing the shape ratio): for instance, a mafic magma with plagioclase (aspect ratio ~4) has a higher viscosity than a similar magma crystallizing olivine (aspect ratio ~2); hence, more mafic melt is needed in the first instance to reach iso-viscous conditions (~10% more, see Supplementary Fig. 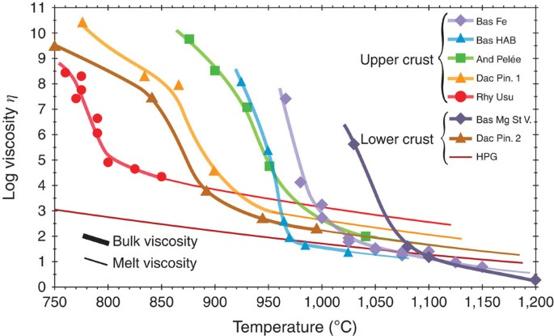3 ). Figure 4: Evolution of magma viscosity with temperature. The melt fraction trends and compositions needed for viscosity calculations are derived from the phase equilibrium works36,44,45,46,47,48,49,50. Melt viscosities (that is, the straight lines in the high temperature part of each curve) differ by <2 orders of magnitude of each other. In contrast, owing to the differences in their temperature interval of crystallization (the mafic composition starting their crystallization at higher temperature than the felsic ones), the viscosity contrast between most felsic–mafic pair (rhyolite-andesite, andesite-basalt or rhyolite-basalt) is often >3 orders of magnitude, except at near liquidus conditions. Bas Fe: Fe-rich basalt49; Bas HAB: high-alumina basalt45; And Pelée: Mt Pelée andesite46; Dac Pin.1: Pinatubo dacite47; Rhy Usu: Usu Rhyolite50; Bas Mg St V: Mg-rich basalt from St Vincent36; Dac Pin. 2: Pinatubo dacite48; and HPG: haplogranite44. Figure 4: Evolution of magma viscosity with temperature. The melt fraction trends and compositions needed for viscosity calculations are derived from the phase equilibrium works [36] , [44] , [45] , [46] , [47] , [48] , [49] , [50] . Melt viscosities (that is, the straight lines in the high temperature part of each curve) differ by <2 orders of magnitude of each other. In contrast, owing to the differences in their temperature interval of crystallization (the mafic composition starting their crystallization at higher temperature than the felsic ones), the viscosity contrast between most felsic–mafic pair (rhyolite-andesite, andesite-basalt or rhyolite-basalt) is often >3 orders of magnitude, except at near liquidus conditions. Bas Fe: Fe-rich basalt [49] ; Bas HAB: high-alumina basalt [45] ; And Pelée: Mt Pelée andesite [46] ; Dac Pin.1: Pinatubo dacite [47] ; Rhy Usu: Usu Rhyolite [50] ; Bas Mg St V: Mg-rich basalt from St Vincent [36] ; Dac Pin. 2: Pinatubo dacite [48] ; and HPG: haplogranite [44] . Full size image Figure 5: Evolution of felsic and mafic magma viscosities with fraction of mafic magma. Viscosities are calculated for an average aspect ratio of crystals, r (given next to each curve) in each magma (see Fig. 3 ), and for the case of a hot mafic magma intruding either shallow ( a , b , c , d ) or deep ( e , f , g , h ) felsic reservoirs. Ticks on curves give the wt% of crystals of each end-member. The upper horizontal axis of each panel is graduated in terms of the SiO 2 (wt%) of the mixture corresponding to the mafic fraction. When the viscosity curves cross over, hybrid magmas are produced. Thick vertical grey lines indicate where the viscosity contrast is <5 (0.3 in log unit). The temperature of each felsic–mafic mixing pair is given by the colour-coded bars. The temperature of the hybrid corresponding to the minimum amount of mafic magma needed to reach near neutral viscosity contrast is given for each case. The initial temperature of magmas in each pair is given in parentheses next to composition. The thin-dashed lines extending the basalt curve on panels a , b and c give the expected bubble effect on viscosity (10% vol). Thick-dashed lines show the viscosity curves of H 2 O-undersaturated felsic magmas. 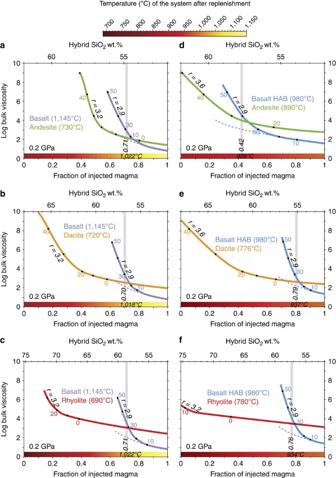Figure 6: Evolution of felsic and mafic magma viscosities with fraction of mafic magma. Viscosity evolution of felsic and mafic magmas are shown for the case of a hot basalt into cold (near solidus) felsic to intermediate reservoirs (a,b,c), and for the case of a cold and wet basalt (HAB, high alumina basalt) into felsic to intermediate reservoirs (d,e,f). Viscosities are calculated for an average aspect ratio of crystals,r(given next to each curve) in each magma. Ticks on curves give the wt% of crystals of each end-member. Thick vertical grey lines indicate where the viscosity contrast is <5 (0.3 in log unit). The temperature of each felsic–mafic mixing pair is given by the colour-coded bars. The temperature of the hybrid corresponding to the minimum amount of mafic magma needed to reach near neutral viscosity contrast is given for each case. The initial temperature of magmas in each pair is given in parentheses next to composition. The thin-dashed lines extending the basalt curve on panelsa,bandcgive the expected bubble effect on viscosity (10% vol). Full size image Figure 6: Evolution of felsic and mafic magma viscosities with fraction of mafic magma. Viscosity evolution of felsic and mafic magmas are shown for the case of a hot basalt into cold (near solidus) felsic to intermediate reservoirs ( a , b , c ), and for the case of a cold and wet basalt (HAB, high alumina basalt) into felsic to intermediate reservoirs ( d , e , f ). Viscosities are calculated for an average aspect ratio of crystals, r (given next to each curve) in each magma. Ticks on curves give the wt% of crystals of each end-member. Thick vertical grey lines indicate where the viscosity contrast is <5 (0.3 in log unit). The temperature of each felsic–mafic mixing pair is given by the colour-coded bars. The temperature of the hybrid corresponding to the minimum amount of mafic magma needed to reach near neutral viscosity contrast is given for each case. The initial temperature of magmas in each pair is given in parentheses next to composition. The thin-dashed lines extending the basalt curve on panels a , b and c give the expected bubble effect on viscosity (10% vol). 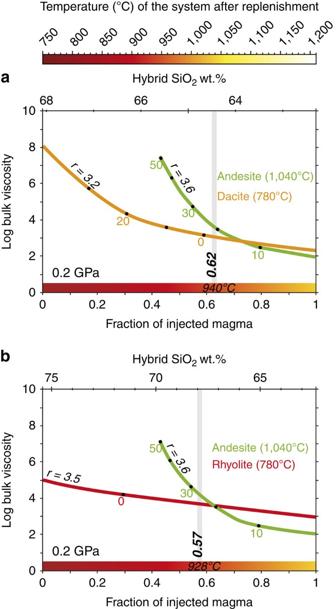Figure 7: Evolution of felsic and intermediate magma viscosities with fraction of intermediate magma. Viscosities evolutions are shown for the case of (a) andesite into dacite, and (b) andesite into rhyolite reservoirs. Viscosities are calculated for an average aspect ratio of crystals,r(given next to each curve) in each magma. Ticks on curves give the wt% of crystals of each end-member. Thick vertical grey lines indicate where the viscosity contrast is <5 (0.3 in log unit). The temperature of each felsic–mafic mixing pair is given by the colour-coded bars. The temperature of the hybrid corresponding to the minimum amount of mafic magma needed to reach near neutral viscosity contrast is given for each case. The initial temperature of magmas in each pair is given in parentheses next to composition. Full size image Figure 7: Evolution of felsic and intermediate magma viscosities with fraction of intermediate magma. Viscosities evolutions are shown for the case of ( a ) andesite into dacite, and ( b ) andesite into rhyolite reservoirs. Viscosities are calculated for an average aspect ratio of crystals, r (given next to each curve) in each magma. Ticks on curves give the wt% of crystals of each end-member. Thick vertical grey lines indicate where the viscosity contrast is <5 (0.3 in log unit). The temperature of each felsic–mafic mixing pair is given by the colour-coded bars. The temperature of the hybrid corresponding to the minimum amount of mafic magma needed to reach near neutral viscosity contrast is given for each case. The initial temperature of magmas in each pair is given in parentheses next to composition. Full size image Altogether, apart from when compositionally similar magmas are mixed (that is, injection of a dacite into rhyolite ( Fig. 5d ), it appears that a significant amount of mafic material (generally >50%) is required to reach small viscosity contrast in upper crustal reservoirs [9] , the resulting mixtures having SiO 2 content in the range 58–55 wt%. For any given felsic–mafic pair, the viscosity curves of each end-member run parallel to each other beyond the crossing point, generally differing by less than one log unit. This suggests that a range of hybrid compositions can be produced beyond the crossing point ( Figs 5 , 6 , 7 ), as observed in many eruptions [6] , [33] . The above reasoning has considered only the mafic into silicic recharge scenario. It has been argued that the reverse situation is common as well [5] . Progressive arrival of felsic magmas into a convecting and hotter mafic reservoir corresponds to a situation much more favourable to efficient mixing, as it implies coexistence of largely (mafic) to fully (silicic) molten end-members ( Figs 5 , 6 , 7 ). Unless there is liquid–liquid immiscibility, such a scenario should end up producing hybrids, provided that the dynamic conditions of the reservoir are favourable [11] . In general, any mechanism able to selectively incorporate, for instance via convective entrainment, small amounts of felsic melt into a mafic magma (thus lying rightward in all panels of Figs 5 , 6 , 7 ) will likely produce hybrids. However, in the common situation of a felsic over mafic layers, such a mechanism remains unclear, as it is the overlying felsic layer, which will convect, thereby entraining underlying mafic parcels. In addition, as further detailed below, such a model cannot explain porphyritic andesites having a significant proportion of phenocrysts inherited from the felsic end-member. As crustal melting is widely believed to occur at the crust–mantle boundary [34] , [35] , [36] , mixing possibilities were also tested at high pressures (0.7–1 GPa), exploring two situations: mixing between basalt and a discrete felsic layer ( Fig. 5e,f ), as would arise from a compaction-segregation process of a partially melted crustal layer [35] , and mixing between basalt and a partially melted, but unsegregated, metamorphic rock ( Fig. 5g,h ). For the first case, the mass fraction of mafic material needed is around 0.7, and hybrids so produced have SiO 2 contents ranging from 55 wt% (dacite layer, Fig. 5e ) to 58 wt% (rhyolite layer, Fig. 5f ). In the second case, a basalt underplating either amphibolite or greywacke crust compositions with no melt segregation at 750 °C requires a mafic mass fraction of at least 0.58 to produce a 54–56 wt% SiO 2 hybrid ( Fig. 5g,h ), which is significantly more viscous, hence less mobile, than when a discrete felsic layer is involved (10 4–5 Pa s versus 10 1–2 Pa s, respectively). Rising the prevailing lower crust temperature to 900 °C decreases to 43–45% the amount of basalt required and produces a 56 wt% SiO 2 hybrid ( Supplementary Fig. 4 ). These calculations thus show that, from the viewpoint of the mass of mafic magma needed, mixing is not facilitated by high-pressure conditions, as everything else being equal (compare b with e and c with f in Fig. 5 ), mixing at higher pressures requires slightly higher proportions of mafic end-member than at low pressure. In other words, hybrid andesites generated in the lower crust will be, on average, more mafic than those produced in the upper crust. For instance, our calculations show that basalt-rhyolite mixing ( Fig. 5c,f ) produce basalt-andesite hybrids in the lower crust (SiO 2 <55 wt%) and true andesites in the upper crust (56 wt%<SiO 2 <58 wt%). As a potential example, Redoubt volcano erupted silicic and mafic andesites, and the latter have been inferred to have been produced at greater depths than those more silicic [51] . It is also remarkable that most hybrids issued from basalt-felsic mixing cluster around 55 wt% SiO 2 , regardless of which felsic end-member (dacite or rhyolite) is being mixed-in. The calculated T-viscosity conditions for the hybrids ( Figs 5 , 6 , 7 ) fall within the field defined by erupted rocks ( Fig. 8 ), those from lower crust showing a trend toward higher viscosities than those produced in upper crustal reservoirs. In detail, andesite hybrids produced from Mg-rich basalt-felsic mixing have temperatures in the range 1,010–1,060 °C, with magma viscosities around 10 2 –10 3 Pa s, whereas andesite hybrids arising from mixing between wet-differentiated basalt and felsic magmas have somewhat lower temperatures (920–940 °C), and slightly higher viscosities, 10 2 –10 4 Pa s ( Fig. 6b ). The crystal content of the former category is 20%, all issued from the mafic end-member ( Fig. 5 ). For the case of wet basalt, the crystal content of the mixture on thermal equilibration is between 20 and 30% ( Fig. 6 ), and apart from when mixing is between basalt and andesite, they are also only of mafic origin. Therefore, an important conclusion, which emerges from these calculations, is that there should be little, if any, felsic-sourced crystals preserved following mixing (excluding the wet basalt-andesite case). This is particularly true for basalt-rhyolite mixing, a common hypothesis for many porphyritic arc andesites [3] , [4] . Hence, a significant part of the crystal cargo of crystal-rich (40–50%) andesites produced by mixing must form after the andesite condition has been reached, that is, during cooling subsequent to mixing. Surviving felsic crystals found in hybrids [3] , in particular quartz and Na-rich plagioclase, most probably relate to the sluggish kinetics of phase dissolution and to the probable causal link between mafic intrusions and eruptions [8] , which arrests mixing phenomena, catching them in the act. 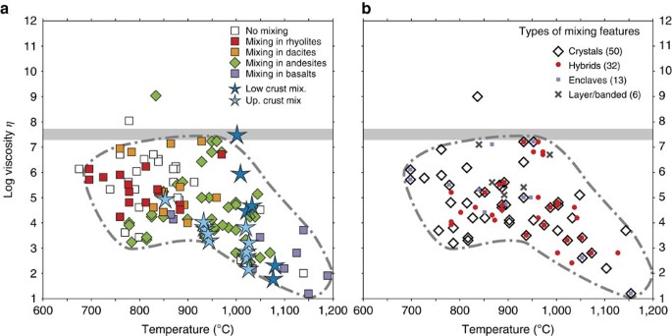Figure 8: Viscosities of natural magmas. (a) Comparison between the pre-eruptive viscosity of volcanic products from the literature27,67,68(squares) and those of hybrids (blue stars) shown onFigs 5,6,7. Colour code indicates the compositional range. Open squares correspond to erupted products bearing no evidence of mixing. (b) For those which have such evidence, the type of mixing texture is shown on panel (b) for each erupted product. The horizontal grey thick line gives the empirical upper viscosity limit beyond which no magma is apparently erupted. Figure 8: Viscosities of natural magmas. ( a ) Comparison between the pre-eruptive viscosity of volcanic products from the literature [27] , [67] , [68] (squares) and those of hybrids (blue stars) shown on Figs 5 , 6 , 7 . Colour code indicates the compositional range. Open squares correspond to erupted products bearing no evidence of mixing. ( b ) For those which have such evidence, the type of mixing texture is shown on panel ( b ) for each erupted product. The horizontal grey thick line gives the empirical upper viscosity limit beyond which no magma is apparently erupted. Full size image Roles of shear rate and bubbles So far, we have assumed that viscosity depends primarily on the crystal load, in addition to crystal shape and melt composition. Other parameters are known to influence viscosity, in particular shear rate [52] and bubbles [53] . To evaluate their role, we use the Pinatubo eruption, a well-known case in which magma mixing has been rigorously documented [32] . Of particular importance in the present context is that, unlike in most instances, end-members before mixing as well as the resulting mixture, are all well characterized, both in terms of composition and P-T-fluid conditions [32] , [47] , [54] . The andesite has been shown to derive from a mixture of 36% basalt-64% dacite, and looks homogeneous at the hand scale [32] . Mixing was achieved in the crustal reservoir where the main dacite body was stored. Calculations show that using pre-eruptive conditions of dacite [47] and pre-intrusion conditions of the basalt [54] , >60% basalt is required to get similar viscosities between end-members ( Fig. 5b ), that is, an amount significantly higher than the true mixture. The simplest way to explain this discrepancy is that the viscosity is affected by either shear rate or bubbles. High shear rates can decrease melt viscosity and promote mixing [11] , [52] . In detail, shear rates associated to enclaves will depend on their mode of formation. Forceful intrusion of basalt into felsic reservoirs may give rise to fountaining, which are associated to local high shear rates [16] . Assuming a fountain height of several hundred metres [16] , a dyke propagation of 0.1−1 m s −1 (ref. 28 ), the calculated shear rates at the interface between a basalt dyke penetrating a cold dacite reservoir are in the range 10 −3 –10 −4 s −1 , that is, comparable to the shear rates needed for the onset of non-Newtonian behaviour (>10 −4 s −1 ). This may well decrease the viscosity contrast down to the field where mixing can operate. In contrast, if enclaves originate from a boundary layer instability [17] , then their rise through the felsic layer will be dictated by the mafic–felsic density contrast. Measurements on quenched enclaves have shown that they preserve a density difference of about −600 kg m −3 with their host [17] . Using typical enclaves sizes (cm to dm (refs 18 , 21 )) their ascent rates predicted by the Stokes law are in the range 10 −5 –10 −7 m s −1 (for a viscosity of 10 5 Pa s, typical of felsic arc magmas [27] ), which correspond to shear rates of 10 −5 –10 −8 s −1 , if the rise occurs over a 1–10-m thick layer (the approximate thickness of a thermal boundary layer [55] ). Such shear rates will not decrease viscosities, and any viscous blob rising through a static felsic layer will likely keep its coherency. However, these ascent rates may be superseded by the vigour of convection in the felsic layer, which is fuelled by the thermal input of the underlying mafic intrusion [55] . Current estimates of convective velocities of felsic reservoirs vary widely [12] , [25] , from 10 −8 m s −1 up to 10 −2 m s −1 , and natural systems quite certainly display a range of convection rates, depending in particular on magma crystallinity. Clearly, stirring velocities at the high end of this range can provide a significant impulse to enclave disaggregation [42] . Turning to bubbles, recent experiments [56] suggest that, under moderate-to-low shear rates, bubbles lead to a drastic decrease in the shear viscosity of magmas: a 10% of volume fraction of bubbles can decrease by up to four orders of magnitude magma viscosity, and such an effect on mixing is illustrated in Fig. 5 . If the basalt replenishing the dacite reservoir coexisted with 10% bubbles (as would occur on its crystallization against the colder dacite [17] ), then the amount of mafic material needed to reach equal viscosities condition is decreased by ~10%, that is, closer to the observed figure. We therefore conclude that both factors (elevated shear rates and bubbles) are indeed facilitators of mixing in shallow reservoirs, and act to decrease the amount of mafic end-member needed to produce hybrids. Accordingly, hybrids resulting from mixing of contrasted magmas (that is, with >10–15 wt% difference in SiO 2 ) and with inferred mafic proportions significantly <50%, suggest either elevated water contents (hence bubbles) or high shear rates, both parameters being possibly interrelated (that is, high volatile contents decrease density hence increase ascent velocities). Even so, preservation of felsic crystals (ex quartz) in any significant proportion seems a rather difficult condition to achieve (see Figs 5 and 6 ). In addition to kinetics effects, armouring of such minerals by newly grown phases [3] may help them withstand dissolution. The role of shear rate and bubbles can be anticipated to be of lesser importance at lower crustal conditions. In particular, owing to the increase in volatile solubilities with pressure, bubble effects in lower crustal mixing processes are likely to be less important. Only CO 2 -rich magmas might be affected, yet the solubility of CO 2 in silicate melts at 1 GPa is>1 wt%, which is higher than dissolved CO 2 contents measured in most melt inclusions, in particular in arc settings [57] . This should further increase the likelihood that hybrids produced in shallow reservoirs are on average more felsic than those originating in the lower crust. Role of magma flux The results above show that to produce an intermediate hybrid rock, a significant amount of mafic magma needs to be injected, broadly as much as the mass of the resident magma ( Figs 5 , 6 , 7 ), which is also similar to that needed to reactivate a large reservoir by remobilization (ca 50 vol.% of mafic magma [58] ). It is worth recalling that most of the cases illustrated in Fig. 5 correspond to largely molten felsic reservoirs. Fully consolidated or near solidus dacitic/granodioritic or rhyolitic-granitic plutons will require much more mafic input, to achieve conditions appropriate to mixing (>80%, Fig. 6 ). We now evaluate if such a situation is viable in natural settings. Hybridization, as modelled in Figs 5 , 6 , 7 , implicitly assumes that the heat exchange occurs between the two end-members only, hence ignores heat loss toward the country rocks. This is equivalent to say that the mafic intrusion is brought rapidly into contact with the felsic reservoir, or at least over a time period during which cooling of the felsic reservoir, owing to conductive heat transfer toward its surrounding, can be neglected. Analyses at various tectonic settings show that long-term magma fluxes are on the order of 10 −3 –10 −4 km 3 yr −1 (ref. 59 ), although considerable variations between and within systems are documented. 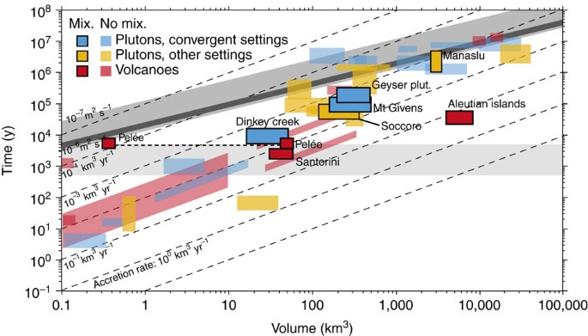Figure 9: Relationships between volumes of reservoir and cooling times. The construction times of intrusive bodies in upper crust60are compared with reservoir solidification times with volume (oblique thick dark curve calculated following59, whereas the lighter-shaded field gives cooling times for two different thermal diffusivities calculated as explained in the main text). Dashed lines give the relationship between average magma flux and reservoir volume. Horizontal shaded field gives the cooling times for dyke thicknesses of 50 and 200 m. The active (molten) part of Mt Pelée reservoir is shown also to the left of full reservoir size69, connected to it by a dashed line. Figure 9 shows the time needed for the assembly of a felsic reservoir in the upper crust, depending on magma fluxes. Also reported are the inferred times of construction for several well-known magmatic systems, either plutonic or volcanic, based on geochronologic and volumetric constraints [60] . This construction time can be compared with the cooling time of each reservoir size (when not fed by mafic input). To estimate the latter parameter, we use the standard diffusion equation: Figure 9: Relationships between volumes of reservoir and cooling times. The construction times of intrusive bodies in upper crust [60] are compared with reservoir solidification times with volume (oblique thick dark curve calculated following [59] , whereas the lighter-shaded field gives cooling times for two different thermal diffusivities calculated as explained in the main text). Dashed lines give the relationship between average magma flux and reservoir volume. Horizontal shaded field gives the cooling times for dyke thicknesses of 50 and 200 m. The active (molten) part of Mt Pelée reservoir is shown also to the left of full reservoir size [69] , connected to it by a dashed line. Full size image where t is time (s), r is reservoir half size (m) and κ thermal diffusivity (10 −7 m 2 s −1 (ref. 59 )). Such an equation assumes that conduction rather than convection is the main mode of heat dissipation of felsic reservoirs, which on the long-term basis is a valid assumption [61] . We first assume the limiting condition of an instantaneous emplacement of a given volume and next consider incremental growth. The characteristic cooling time of a spherical reservoir is shown superimposed on reservoir construction time of Fig. 9 (depending on a particular flux rate of magma). For each flux rate, any reservoir size plotting below the cooling curve is still fully or partially molten. Hence, if intercepted by an ascending mafic batch, it will be prone to hybrid production, provided the supplied amount of mafic magma is broadly equivalent to that of the resident magma (or the part, which is still molten), in accordance with constraints from Figs 5 , 6 , 7 . Conversely, any system lying above the cooling curve will be essentially solid, and unable to mix with mafic forerunners. For an average magma flux rate of 10 −3 km 3 yr −1 , system volumes lower than 1,000 km 3 remain liquid, whereas for a flux rate of 10 −4 km 3 yr −1 , the critical volume beyond which the reservoir will be frozen is significantly smaller, <1 km 3 . The geological trend crosses the cooling curve at the high end, which would suggest that mixing operates in almost all circumstances, with the implication that large volumes of hybrids can be achieved by mixing in upper crust. However, for the more likely scenario of incremental growth of plutons [37] , [38] , the cooling pattern is dictated by the size of sill intrusion as well as by the time interval between two successive magma additions. In such a case, numerical simulations [37] , [38] have shown that at flux rates lower than 10 −3 –10 −2 km 3 yr −1 , no molten reservoir of any significant size can develop, which considerably restricts the likelihood of widespread efficient mixing in upper crust. Each individual sill (thicknesses of 50–200 m) will cool down solidus in <500–5,000 years, which truncates the natural trend at reservoir volumes of about 10–100 km 3 ( Fig. 9 ). At an average rate of 10 −4 km 3 yr −1 , incubation time needed to start accumulating melt in mid-sized reservoirs (10–100 km 3 ) are in the range 60–120 k yr (ref. 37 ), beyond which only 10% of the intruded mass remains active (that is, partly molten, see the case for Mt Pelée Fig. 9 ). This indicates that, in upper crust, mixing will potentially have a petrogenetic role during the late stage of pluton construction, and affect a small part only of the whole intrusion. Hence, large reservoirs built in upper crust at average flux rates lower than 10 −2 –10 −3 km 3 yr −1 will be unfavourable locii to the production of hybrid rocks in any significant amounts, instead preserving abundant evidence of magma blending and incomplete mixing [28] , [29] , [30] (that is, mingled magmas). This rule, however, may be violated whenever a surge in magma-feeding rates happens during batholith construction [37] , [62] . Note that mixing needs not to involve all the mass of felsic magma. Beside the above thermal restrictions, the fluid dynamics associated to reservoir recharge may restrict efficient mixing to a small portion of the intruded reservoir as illustrated by the Pinatubo eruption [63] . The previous arguments show that hybrids require above all vast amounts of mafic magmas (relative to felsic) being injected rapidly into partially molten felsic reservoirs. Therefore, when rooted into magmatic systems of inferred small dimensions, emission of abundant hybrid andesites bears witness of enhanced magmatic production along with that particular mantle–crust section. Systems characterized by relatively low magma fluxes will, in contrast, produce bimodal magmatic provinces, if mixing is the main driver of magma compositional diversity. Recent modelling studies have concluded that magmatic bimodality is favoured by volatiles-poor magmas and low-heat input [36] . The present work reinforces and adds a rheological dimension to such a paradigm, showing that low-heat input and bubble-free regime inhibit efficient small-scale homogenization, thus preserving magma diversity. From a volcanological perspective, the demonstration that most crystals of the felsic end-member should melt out on mixing provides a robust time scale on mixing phenomema in eruption contexts. Preservation of felsic phenocrysts shows that thermal excursions associated to magma intrusion are highly transient. For instance, experiments on Pinatubo dacite show that complete melting of H 2 O-rich dacite at 930 °C takes place in a day or so [47] , which provides an upper bound on the time spent between basalt intrusion and andesite eruption for this particular case. The fact that mixing is not enhanced at high pressures suggests that magmas produced in the deep crust may well preserve its chemical heterogeneity. Intermediate to felsic magmas derived from lower crustal processes are thus likely to be faithful mirrors of lower crustal lithologies at regional scales at least [7] . However, any sizeable mass of rock, demonstrably hybrid in origin, must have been produced in the deep crust before emplacement in upper crust, owing to the severe thermal restrictions imposed on mixing efficiency by the mechanism of incremental growth at shallow levels. At last, the pressure effect has also implications for the understanding of the chemical evolution of the continental crust. A thin crust frequently intruded by hot basalt, as could have been the case in the early Earth, has the potential to produce large amounts of relatively felsic hybrids. Conversely, an increase in crust thickness, correlated to a lower mantle heat flux, are bound to produce less, but more mafic, hybrids, and thus drive the bulk composition of the continental crust toward a more mafic composition. This may have helped to produce an Archean continental crust more silicic than the Phanerozoic one [64] , as there are no reasons to believe that mixing was a less important petrogenetic mechanism in the Archean than nowadays. Starting materials Samples for torsion experiments were composed of pairs of magmas from the three starting materials whose compositions are given in Supplementary Table 1 . The most felsic end-member is a synthetic haplotonalite manufactured by Schott A.G. (Germany), which has been extensively used in previous deformation experiments [65] . Its composition allows the crystallization of plagioclase ~An 30 only over a large range of crystal fraction (0–65% in volume) and temperature (~700–1,220 °C) depending on water content. In the first series of experiments, the magma juxtaposed to the haplotonalite was a natural dacite of Santorini Volcano (Greece), which was previously melted at 1 bar at 1,500 °C to produce a crystal-free dacite glass. The mafic end-member of the second and third series of experiments was a basalt from a lava flow from Santorini Volcano: this starting basalt is holocrystalline and was used directly in the torsion experiments. Syntheses of starting material In the first series of experiments, both compositions (haplotonalite and dacite) were melted at 1,500 °C for 3 h in a 1-atm furnace to get dry, crystal-free, magmas. The water content in both melts is lower than 0.1 wt% and no crystals were detected. After the torsion experiments, both magmas remained free of crystals, except the dacite in the experiment conducted at 1,000 °C (see below), which displayed a 20-μm thick crystallized halo at the interface with the haplotonalite. The second series of experiments involved the crystal-bearing basaltic magma, together with the same dry, crystal-free, haplotonalite used in the first series. Both magmas were used dry in an effort to limit quench phases. The haplotonalitic magma remained crystal-free at T <1,150 °C, but started to crystallize at the highest temperatures investigated (1,150–1,200 °C), producing a thin halo at the interface with basalt or capsule (<150 μm) for the longest experimental durations (~8 h). The crystallization interval of the basalt ranges between ~1,000 and 1,230 °C and the run temperature was adjusted to produce different viscosity contrasts between end-members. See Laumonier et al. [66] for a detailed description of the textures and chemical compositions of the phases in the starting materials and experimental products. The third series of experiments used hydrous crystal-bearing haplotonalite and basalt glasses, which were obtained by a first crystallization experiment at P =300 MPa, T =950/1,000 °C, t =7 days in an internally heated pressure vessel. This first stage produced water-saturated crystal-bearing melts with 38 and 53% (950 °C) and 31 and 45% (1,000 °C) of crystals for the felsic and the mafic components, respectively. The syntheses performed at 950 °C were used in torsion experiments conducted at 600, 715, 950, 975 °C, whereas that at 1,000 °C was used in torsion experiments performed at and 985, 1,000, 1,020 °C. The crystal contents of first-step syntheses were preserved in the torsion experiments conducted at 600 and 715 °C. For other deformation experiments, small changes in crystal content occurred, toward either higher (that is, a torsion experiment at 985 °C using a synthesis at 1,000 °C) or lower proportions depending on whether the temperature of mixing experiment was higher or lower than that of the first-step synthesis temperature. These small changes in phase proportions were taken into account in the viscosity calculations, using a melt fraction versus temperature relationships calibrated experimentally for each composition. Deformation experiments Torsion experiments were conducted in a Paterson apparatus [39] at 300 MPa, strain rates ranging from 3 × 10 −5 to 3 × 10 −3 s -1 , and various temperatures ( Supplementary Tables 2–5 ). During torsion experiments, the torque of the assembly containing the sample was recorded. Then, the torque was corrected from the jacket contribution to calculate the shear stress and the viscosity of the sample only [39] . The error on viscosity calculation depends on the intrinsic precision of the load cell recording the internal torque, on the regularity of the plateau that defines the value of the torque and on the jacket contribution. The maximal theoretical error on the viscosity was calculated by adding all three factors and is listed in Tables 2–5 and in Fig. 2 (see main text). Two kinds of samples were prepared depending on the target of the experiment. To characterize the rheological evolution of end-members with temperature, the cylindrical sample inserted into the Paterson press was composed of a single layer of that end-member (dry, crystal-free dacite and haplotonalite and dry, melt-bearing basalt) whereas to investigate the mixing capacities between two magmas, the samples consisted in a stack of 2–4 layers alternating in composition ( Supplementary Fig. 1 ; see also ref. 66 ). When a torsion deformation is applied to either a two- or four-layers stack ( Supplementary Fig. 1 ), it imparts simple shear along the various interfaces between compositionally different layers (if their rheological properties differ). This shearing mechanism is similar, for instance, to that occurring at the interface between a rising basaltic dyke into a felsic reservoir, or between a basaltic sill flowing at the base of a felsic reservoir and its felsic host. Viscosity calculations In addition to direct viscosity measurements performed with the Paterson press, we calculated the expected magma viscosities at our P-T conditions. Melt viscosity η melt was calculated using the model of ref. 40 . The effect of crystals, that is, the relative viscosity η rel , depends on both the crystal fraction ( φS ) and the shape ratio ( r ) of the crystals. In this study, we derived an empirical model to calculate the relative viscosity η rel, by combining several models and published (see Supplementary Table 6 ) and unpublished data ( Fig. 3 ). This model is restricted to a crystal fraction lower than 0.6, and assumes that several crystal populations with different shape ratios can be considered as a unique population with an average shape ratio r . The empirical equation fitting the available data is: with α =0.373 × r +4.89, β =17.241 × exp 0.748· r , ϕ =−3.96 × r , δ =0.108 × r −0.292, ε =2 × 10 −4 exp 3.50· r , ζ =−24 × r +52.6. Injected fraction of mafic magma and viscosity Input parameters used to calculate the final temperature reached by a system composed of a felsic reservoir replenished by a mafic intrusion are given in Supplementary Tables 7,8 . The calculations were done using the method of ref. 9 . The initial temperature of each mafic magmas was its liquidus temperature. The initial temperatures of the felsic end-members were chosen to encompass the pre-eruptive temperatures of felsic reservoirs in arc settings [27] , except for the case of the melting of lower crust lithologies (see Supplementary Table 8 ). How to cite this article: Laumonier, M. et al. On the conditions of magma mixing and its bearing on andesite production in the crust. Nat. Commun. 5:5607 doi: 10.1038/ncomms6607 (2014).